Cold ablation driven by localized forces in alkali halides Laser ablation has been widely used for a variety of applications. Since the mechanisms for ablation are strongly dependent on the photoexcitation level, so called cold material processing has relied on the use of high-peak-power laser fluences for which nonthermal processes become dominant; often reaching the universal threshold for plasma formation of ~1 J cm −2 in most solids. Here we show single-shot time-resolved femtosecond electron diffraction, femtosecond optical reflectivity and ion detection experiments to study the evolution of the ablation process that follows femtosecond 400 nm laser excitation in crystalline sodium chloride, caesium iodide and potassium iodide. The phenomenon in this class of materials occurs well below the threshold for plasma formation and even below the melting point. The results reveal fast electronic and localized structural changes that lead to the ejection of particulates and the formation of micron-deep craters, reflecting the very nature of the strong repulsive forces at play. Laser ablation involves many-body interactions which, in a collective response to optical excitation, lead to material removal. The ablation processes in metals, semiconductors and dielectrics are different owing to the nature of their electronic and structural properties. In the case of semiconductors and metals exposed to femtosecond (fs) laser irradiation, different absorption energy regimes have been observed [1] , [2] , [3] , [4] . At relatively low incident laser fluence ( F <100 mJ cm −2 ), the solid surface is heated up and the material thermally evaporates or sublimes on the nanosecond-to-microsecond timescale. At higher laser peak powers, providing F is in the range of 300–500 mJ cm −2 , the system is often pushed into a metastable liquid phase as a result of rapid heating and melting. In such a metastable state, homogeneous bubble nucleation leads to the removal of large fragments of the material through processes known as spallation, phase explosion and fragmentation [5] , [6] . With even higher F (>1 J cm −2 ), the solid surface changes directly into a gaseous plasma via multiphoton ionization. This often leads to the ejection of charged fragments due to strong space-charge effects [7] . This latter process, which involves states that are unreachable by any possible thermal pathway, is commonly referred to as ‘cold ablation’ and relies on effective potential energy channelling into translational degrees of freedom. Due to their much wider bandgap ( E g ), fs laser interaction with dielectrics often involves multiphoton absorption processes. If E g largely exceeds the photon energy ( hν ), absorption is frequently dominated by highly nonlinear processes that lead to ionization and avalanche effects [8] , [9] , [10] . The investigation of elementary electron–hole pairs (excitons) in ionic dielectric materials, such as alkali halides, has therefore required the use of hv in the ultraviolet (UV) range to mitigate the aforementioned competing channels. The effects of UV light on the electronic properties of alkali halides were discovered in 1896 when initially colourless crystals were found to gain colour on irradiation [11] . Since then, several studies have been performed to understand the formation of such long-lived colour centres [12] . By analogy to gas phase studies [13] , the observed absorption band in alkali halides was initially attributed to the electron back transfer from the anion to a neighbouring cation. In this case, the cation would gain neutral character and thus absorb light in the visible range of the spectrum. The scenario in the crystalline phase was found to be considerably more complicated than that for contact ion pairs in vacuum, with different species originating from a highly unstable primary exciton. Nevertheless, the highly localized nature of the excited state in alkali halides made these materials an ideal target for the investigation of self-trapped excitons, self-trapped holes and different transient precursors of long-lived lattice defects and vacancies responsible for the chromatic effect [14] , [15] , [16] , [17] , [18] , [19] , [20] , [21] . Moreover, several experiments involving time-resolved ion detection have been performed to investigate the stability of alkali halide surfaces following fs laser irradiation [22] , [23] , [24] , [25] at moderate F ~1–10 mJ cm −2 or low-energy electron irradiation [26] . These results have connected the states of alkali halides irradiated by fs laser pulses or electron beams with surface desorption mechanisms. In these studies, surface metallization [25] and nonthermal layer-by-layer [26] desorption processes, driven by the formation of excitons, have been proposed. On the other extreme, the ablation process due to Columbic explosion induced by multiphoton ionization of the sample’s surface has also been discussed for dielectric materials at very high photoexcitation levels [27] , [28] , F >1 J cm −2 . In this report, we investigate the mechanism and driving force of the ablation process that follows 2 or 3 photon fs laser excitation of alkali halides under the intermediate range of photoexcitation F ~100 mJ cm −2 . This range has not been fully explored and it is critical to separate novel electronic factors related to Pauli repulsion forces from multiphoton ionization effects. We performed single-shot fs electron diffraction (FED) to track the structural changes associated with laser-driven lattice disruption in this critical fluence regime. This information is complemented by fs optical reflectivity to fully resolve the dynamics and by ion detection studies to link bulk structural and electronic changes to the nature of the ablation process. Our results provide clear evidence of the fast optical and structural changes in alkali halide materials, indicating the development of a lattice-disordering process followed by the expulsion of large clusters and/or fragments. We found that fragmentation remains quite significant even at the moderate laser fluences. For instance, half-a-micron-deep craters are formed in polycrystalline KI sample using single 400 nm pulses with a fluence value of 60 mJ cm −2 . The amount of absorbed energy (2–4% of the incident) is insufficient in this case to melt the sample, confirming the nonthermal character of the ablation mechanism. Fs optical reflectivity and ion detection in silicon We present our results alongside time-dependent reflectivity changes and ion detection measurements obtained for Si, chosen as a reference system because its fs laser melting and ablation processes are well characterized [29] , [30] , [31] , [32] , [33] , [34] , [35] . Thermal melting for Si is expected to occur for F in the range of 35–70 mJ cm −2 , which shows up as an increase in reflectivity during the first ~5 ps (black traces in Fig. 1a ) owing to the onset of metallic character caused by the formation of liquid Si [36] . Laser fluences of 70–100 mJ cm −2 correspond to about 9% of valence carrier excitation and are known to trigger a much faster nonthermal disordering process that takes place on a timescale of 200–400 fs [36] , [37] , [38] , [39] , [40] , [41] . This effect correlates with a very sharp increase in reflectivity observed in the sub-500 fs temporal span (red trace in Fig. 1a ). The decrease in reflectivity occurring on the 100 ps timescale is due to surface removal caused by ablation processes that correspond to the spallation, phase explosion and fragmentation of the material. A similar response, which is more pronounced in terms of reflectivity changes, is observed [42] , [43] , [44] for F higher than 200 mJ cm −2 (see blue and magenta traces in Fig. 1a ). This latter observation correlates with the first ablation threshold, F abl , determined in our ion detection measurements (see Fig. 2a ). For F > F abl ≈200 mJ cm −2 , the detection of positively charged fragments from Si is evident. There is in general good agreement between our time-resolved reflectivity and ion detection measurements, and previous studies [30] on laser-induced surface disordering of Si. As shown in Fig. 2a , increasing the incident fluence above 800 mJ cm −2 results in a dramatic enhancement of the ion yield. This new threshold fluence, F plasma , was attributed to the formation of gaseous plasma. According to the literature [44] , this process becomes dominant at F >1 J cm −2 . In summary, we have found, through ion detection measurements, two ablation thresholds ( F abl ≈200 mJ cm −2 and F plasma ≈800 mJ cm −2 ) for Si that concur with previous findings [34] , [35] , [42] . 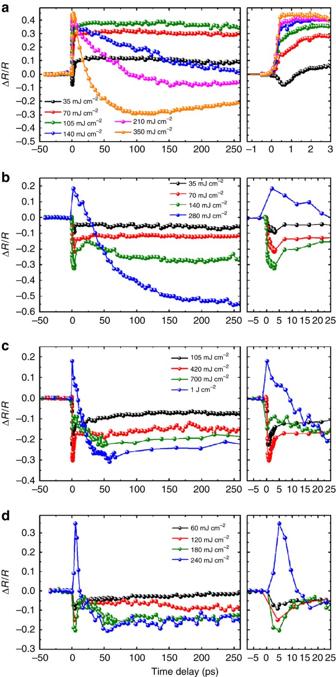Figure 1: Time-dependent reflectivity changes. Relative reflectivity changes as a function of the time delay (a) for Si, (b) for CsI, (c) for NaCl and (d) for KI. The incident laser fluences corresponding to the each plot are indicated in the figures. Figure 1: Time-dependent reflectivity changes. Relative reflectivity changes as a function of the time delay ( a ) for Si, ( b ) for CsI, ( c ) for NaCl and ( d ) for KI. The incident laser fluences corresponding to the each plot are indicated in the figures. 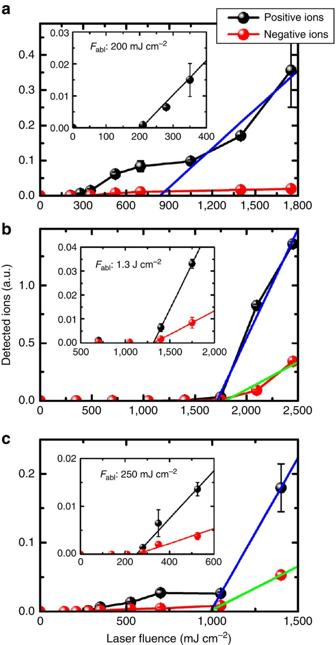Figure 2: Ablation ion yields as a function of laser fluence. Laser fluence-dependent yields of positive (black trace) and negative (red trace) ions measured using a simple homemade ion detection system (a) for Si, (b) for NaCl and (c) for CsI single-crystalline samples. Insets show magnified views near the first detected ablation threshold,Fabl, for each sample. The second threshold,Fplasma, is determined as the intersection of the blue and/or green lines with the abscissa. The difference in the yield of negative and positive ions reflects the fact that, in general, cations are more thermodynamically stable species than their corresponding anions. Full size image Figure 2: Ablation ion yields as a function of laser fluence. Laser fluence-dependent yields of positive (black trace) and negative (red trace) ions measured using a simple homemade ion detection system ( a ) for Si, ( b ) for NaCl and ( c ) for CsI single-crystalline samples. Insets show magnified views near the first detected ablation threshold, F abl , for each sample. The second threshold, F plasma , is determined as the intersection of the blue and/or green lines with the abscissa. The difference in the yield of negative and positive ions reflects the fact that, in general, cations are more thermodynamically stable species than their corresponding anions. Full size image Fs optical reflectivity and ion detection in alkali halides Owing to the wide bandgaps of CsI (6.1 eV), NaCl (7.6 eV) and KI (6.0 eV) crystals, photoexcitation with 400-nm wavelength light (3.1 eV) requires two or three photons for above bandgap excitation and the creation of electron–hole pairs. The time-dependent changes in reflectivity for CsI and NaCl single crystals and polycrystalline KI films, presented as black and red curves in the Fig. 1b–d for the range of modest F , exhibit a sharp sub-picosecond decay in amplitude, followed by a partial recovery with several picosecond rise times. This trend is clearly different from the rapid enhancement in reflectivity followed by its subsequent decay within 100–200 ps observed for the Si ( Fig. 1a ) under similar photoexcitation conditions. At F ≈140, 700 and 180 mJ cm −2 , for Fig. 1b–d , a small bump appears at the end of the well in the green traces shown for CsI, NaCl and KI, respectively. Going to even higher fluences makes this feature grow (blue traces in Fig. 1b–d ) into a large peak closely resembling that observed during the formation of liquid Si. On the basis of the fact that the reflectivity of ionic and glass materials increases as they melt [45] , the latter result provides strong evidence for melting occurring at the crystal’s surface. Therefore, we can consider those values of F , 140, 700 and 180 mJ cm −2 , as an estimate for the onset of thermal melting, F melt , for CsI, NaCl and KI samples, respectively. On the other hand, it is safe to assume by inspecting the red traces in Fig. 1b–d that no melting happens for the corresponding alkali halides at and below the 70, 420 and 120 mJ cm −2 fluences. The ion detection measurements for NaCl and CsI samples are summarized in Fig. 2b,c . Through careful examination of the CsI data, we also found a two-threshold behaviour with F values of ≈250 mJ cm −2 and ≈1 J cm −2 for ion detection, which are higher than F melt . In direct comparison with the Si data, the former threshold can be related to spallation, phase explosion and fragmentation processes. The latter threshold is assigned to gaseous plasma formation. In the case of NaCl, these two thresholds are very close, F abl ≈1.3 J cm −2 and F plasma ≈1.7 J cm −2 , suggesting that both processes might occur near-simultaneously or that ionization effects leading to plasma formation are simply dominant due to its relatively higher ratio. 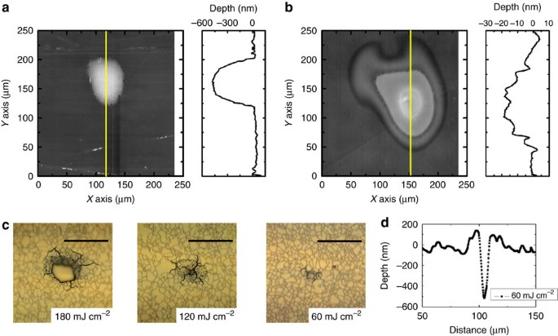Figure 3: Crater measurements. All craters were produced by single 400 nm pump pulses. Micrographs of the craters alongside their 2D sectional profiles for single-crystalline CsI (a) and single-crystalline Si (b); incident fluences were 140 and 350 mJ cm−2, respectively. (c) Craters generated in 2.5-μm-thick polycrystalline KI films atF≈60–180 mJ cm−2(scale bar, 100 μm). (d) Representative profile measurements for the crater shown inc,F≈60 mJ cm−2. Crater depth measurements Figure 3a,b shows typical crater shapes observed via optical interferometry after exposing CsI and Si samples to single-excitation pulses with F =140 and 350 mJ cm −2 , respectively. The crater profiles in KI ( Fig. 3c ) and NaCl samples were measured with a stylus contact profilometer and confocal laser microscopy. A brief summary of the crater depths obtained for each sample with various laser fluences is presented in Table 1 . Overall, KI samples retain the highest crater depth among all studied alkali halides, with its value being nearly 100 times larger than that in Si owing to the fundamental difference between fs laser ablation of semiconductors and dielectric materials [9] . We would like to emphasize here that the result of producing larger craters in KI when compared with CsI and NaCl is readily anticipated. Polycrystalline samples are composed of small crystallites with weaker inter-crystallite forces, and therefore are softer than the single-crystalline counterpart. What is interesting though are the unusually deep (≈0.5 μm) craters created in alkali halides using single laser pulses with F < F melt < F abl <F plasma . For comparison, making a similar size crater in Al 2 O 3 with a single laser shot requires nearly two orders of magnitude higher flux with F =11.3 J cm −2 for 395 nm light [46] . Another important point is the mechanism responsible for the material expulsion. It is definitely nonthermal in nature, since according to our results no sample melting should happen. Figure 3: Crater measurements. All craters were produced by single 400 nm pump pulses. Micrographs of the craters alongside their 2D sectional profiles for single-crystalline CsI ( a ) and single-crystalline Si ( b ); incident fluences were 140 and 350 mJ cm −2 , respectively. ( c ) Craters generated in 2.5-μm-thick polycrystalline KI films at F ≈60–180 mJ cm −2 (scale bar, 100 μm). ( d ) Representative profile measurements for the crater shown in c , F ≈60 mJ cm −2 . Full size image Table 1 Summary of crater depth measurements. Full size table It has been proposed that nonthermal fs laser ablation in dielectric materials proceeds through surface charging, followed by impulsive Coulomb explosion [28] . However, the experimental conditions in this work are significantly different from those in the aforementioned studies for single-shot ablation (800 nm, 200 fs, 5 J cm −2 ). We cannot therefore explain our findings for large crater formation in alkali halides with this mechanism, as the low laser fluences used in the current experiments are far insufficient ( F ≪ F plasma ) to generate the required charge density for Coulomb explosion to take off. FED measurements To further elaborate on the nonthermal mechanism of the ablation process, we performed single-shot FED experiments providing direct structural information on the evolution of crystalline order following fs photoexcitation. 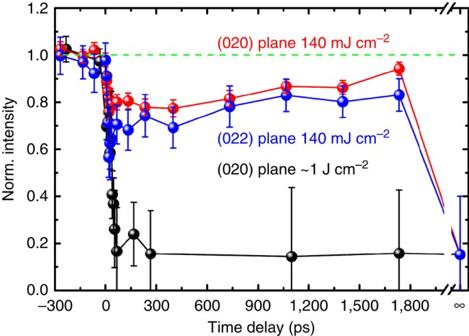Figure 4: FED measurements. Time-dependent changes in electron diffraction intensity for KI under non-reversible, single-shot photoexcitation conditions. Red and blue traces correspond to the relative changes observed for (020) and (022) Bragg reflections, respectively, atF≈140 mJ cm−2. Black trace corresponds to relative changes for the (020) reflection atF≈1 J cm−2. Vertical error bars represent one s.d. from the mean values for the changes in electron diffraction intensity. Due to irreversible sample damage, the statistics is limited to either 8–10 (blue and red data points) or 5 (black and infinity time data points) single-shot measurements. The green dashed line is a no-change-in-diffraction-intensity guide to the eye. Norm., normalized. Figure 4 shows the time-dependent diffraction intensities for the (020) and (022) Bragg reflections from 50-nm-thick ‹100›-oriented KI films photoexcited with 400 nm light. The red and blue traces ( F =140 mJ cm −2 ) in Fig. 4 reveal the decrease in the crystalline order during the first few tens of picosecond, which then recovers gradually on the nanosecond timescale. The electron diffraction data can be used to estimate the lattice temperature of the KI sample after fs laser irradiation. Accordingly, the recorded intensity signal from diffracted electrons ( I ) can be expressed by the following equations: Figure 4: FED measurements. Time-dependent changes in electron diffraction intensity for KI under non-reversible, single-shot photoexcitation conditions. Red and blue traces correspond to the relative changes observed for (020) and (022) Bragg reflections, respectively, at F ≈140 mJ cm −2 . Black trace corresponds to relative changes for the (020) reflection at F ≈1 J cm −2 . Vertical error bars represent one s.d. from the mean values for the changes in electron diffraction intensity. Due to irreversible sample damage, the statistics is limited to either 8–10 (blue and red data points) or 5 (black and infinity time data points) single-shot measurements. The green dashed line is a no-change-in-diffraction-intensity guide to the eye. Norm., normalized. Full size image and Where K is the scattering vector, F ( K ) is the structure factor, G ( K ) is the Laue function, f j ( K ) is the atomic scattering factor, D j ( K ) is the Debye–Waller factor and r j is the equilibrium position of the j th atom in the unit cell. The Debye–Waller factor can be written in terms of temperature-dependent B -factors ( B j ) or through the mean square displacement ( U j ) as where θ is the scattering angle and λ is the de Broglie wavelength of the electrons. We performed a temperature analysis based on values of B -factors obtained from the parameterization in ref. 47 derived from the experimental phonon density of states data (see Supplementary Note 1 for more details about these calculations). Assuming the largest intensity change of 25 and 45% for the (020) and (022) Bragg reflections from 140 mJ cm −2 data in Fig. 4 , the predicted lattice temperature is ≈1,200 K (kinematic diffraction theory) or ≈1,800 K (with corrections from dynamical diffraction theory [48] ). These lattice temperatures are certainly above the melting point, and therefore fall off the validity range of the Debye–Waller model, which is only applicable if the unit cell structure of the crystalline material remains intact. After the slow recovery of the signal (time delays of ≈1–2 ns), Debye–Waller analysis predicts a T l =725±110 K that is below the melting point of the salt, 954 K. It is worth mentioning that by comparison (see Supplementary Figs 1 and 2 ), 100-nm-thick KI films show a much stronger intensity decay than those observed for 50-nm-thick films. A similar attenuation effect on the electron diffraction intensity for all diffraction orders was found to be dependent on the material thickness [49] . Accounting for this effect in the analysis results in a smaller temperature increase. Therefore, the observed drop in intensity for the (000)-order electron beam implies that our predicted increase in lattice temperature is indeed an upper estimate. Despite the limitations of the analysis of the FED data, the above findings support the fact that sample heating is insufficient by itself to explain the observed changes in the diffraction, suggesting there are other processes related to the loss and recovery of crystallinity that are occurring in parallel. One of the possible mechanisms leading to the lattice damage is the formation of point defects in the crystal from self-trapped excitons [20] . The effect of vacancy concentrations on diffraction signal from nanocrystalline materials was previously investigated [50] . On the basis of those predictions, it would require more than 20% (≈2 × 10 21 cm −3 ) lattice point defects to decrease the (020) diffraction intensity by 25%. Such high concentration of point defects is not reachable in our study, which is evident from the optical measurements showing that there are <10% photoexcited halide centres at F= 140 mJ cm −2 (see Supplementary Note 2 for the details). The other viable causes for the loss of crystallinity are partial local disordering or melting. Referring to the optical reflectivity measurements in KI, F= 140 mJ cm −2 falls into the 120–180 mJ cm −2 interval that loosely defines the melting threshold. As a result, when the incidence laser fluence is in close proximity to that of F melt , there is a high probability that a fraction of the sample locally becomes either significantly disordered or turns into a liquid. Most likely, in addition to the sample heating, local disordering is the key factor responsible for the reduction in diffraction signal. As the temperature of the sample starts equilibrating within the photoexcited volume, these highly disordered regions attempt to recrystallize, thus contributing to the slow recovery in the diffraction intensity observed in a nanosecond time interval. The latter conclusions are also supported by time-resolved diffraction data at F =1 J cm −2 (shown in Fig. 4 ). No signal recovery is detected for the plasma-driven damage in KI at this level of fluence. Following energy conservation, the increase in lattice temperature after photoexcitation can also be estimated as where A eff is the effective absorbed fluence fraction, f t is the film thickness ~50 nm, ρ and C are the material’s density (3.12 g cm −3 ) and specific heat capacity (313 J kg −1 K −1 ) for KI, respectively. In a very conservative scenario that considers A eff ≤ 4% (see Supplementary Fig. 3c ), equation (4) provides Δ T l ≤ 1,150 K. Since the sample was originally at room temperature, the lattice temperature after thermal equilibration therefore results in ( F =140 mJ cm −2 ) ≤1,440 K. Despite the fact that the calculated value of is an upper estimate, crater formation in KI was found to occur at F as low as 60 mJ cm −2 (see Table 1 and Fig. 3c ) for which equation (4) would predict ( F =60 mJ cm −2 ) <780 K, which is below the melting point. A similar conclusion can be drawn for NaCl modifying equation (4) by replacing f t by d c (the crater depth) and A eff by the absorbed fraction measured across the 2-mm-thick bulk single crystal. Hence, a simple thermodynamic calculation based on upper estimates for the absorbed energy, which is in agreement with the values of F melt determined via fs optical reflectivity measurements, provides strong evidence for nonthermal pathways to be the dominant driving force for the ejection of particulates. The forces involved can be understood through a simple analogy with contact ion pairs in the gas phase ( Fig. 5a ). Optical excitation induces localized changes in the electronic distribution, that is, strong electronic stress [51] , [52] , [53] , [54] , [55] that provides the initial kick for the consequent material ejection. This latter explanation is consistent with the observation of strain waves [56] in the GHz range (see oscillatory behaviour in fs optical reflectivity data shown in Supplementary Fig. 4 ). A strongly localized nature of the excited state is also supported by the FED data (red and blue traces in Fig. 4 ), which give evidence for the creation of disordered regions that release their energy to the surrounding unexcited crystal (recovery of diffraction signal on sub-ns timescale). At systematically higher fluences necessary to invoke substantial ablation, ion detection thresholds indicate that the sample is likely ejected in the form of large clusters and/or particulates, provided the yield of relatively high (up to 4,000) ions being emitted from the irradiated alkali halide crystals. Such behaviour is common for the fs laser ablation of dielectrics and has been extensively used in industry for pulsed-laser deposition of thin films [9] . The long time scales for the material expulsion in alkali halides nicely correlate with the slow speed of the nanosized particles. However, the assumption about plume composition has to be verified by future experiments. 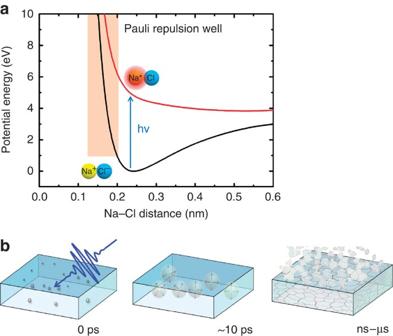Figure 5: Summary of cold ablation process. (a) Calculated potential energy curves for the NaCl molecule. The ionic ground and neutral excited states are plotted as black and red curves, respectively (for more details see Computational method Section). Vertical excitation brings the system right to the onset of the Pauli repulsion well where short-range core–core repulsion forces are dominant. The core–core repulsion forces are also expected to be one of the key factors responsible for the material expulsion in alkali halide crystals68. (b) A pictorial representation of the cold ablation process. Similar to the NaCl molecule, photoexcitation in alkali halide crystals causes a local change in the electronic density around the excited halide anions and their neighbouring alkali cations, thus unleashing repulsive forces between partially neutralized atoms. To release the stress, pertinent atoms move from their ground state equilibrium positions and form disordered regions within several picoseconds after the photoexcitation. Further relaxation of the lattice, subject to the amount of generated strain, might involve cracking and ejection of the material on the nanosecond-to-microsecond timescales. Figure 5: Summary of cold ablation process. ( a ) Calculated potential energy curves for the NaCl molecule. The ionic ground and neutral excited states are plotted as black and red curves, respectively (for more details see Computational method Section). Vertical excitation brings the system right to the onset of the Pauli repulsion well where short-range core–core repulsion forces are dominant. The core–core repulsion forces are also expected to be one of the key factors responsible for the material expulsion in alkali halide crystals [68] . ( b ) A pictorial representation of the cold ablation process. Similar to the NaCl molecule, photoexcitation in alkali halide crystals causes a local change in the electronic density around the excited halide anions and their neighbouring alkali cations, thus unleashing repulsive forces between partially neutralized atoms. To release the stress, pertinent atoms move from their ground state equilibrium positions and form disordered regions within several picoseconds after the photoexcitation. Further relaxation of the lattice, subject to the amount of generated strain, might involve cracking and ejection of the material on the nanosecond-to-microsecond timescales. Full size image In summary, we found evidence for a cold laser ablation process that takes place in alkali halides upon photoexcitation of only a few percent of the halide centres. The observed dynamics illustrates the very nature of highly localized repulsive forces involved in the ejection of material. As computing power grows and different simulation tools are developed [57] , ab initio molecular dynamics will be able to provide a more detailed microscopic understanding of this cold ablation process. Single-shot FED measurements Time-resolved electron diffraction measurements have been performed in transmission mode to minimize the effects of surface charging, which can dominate the behaviour of the electron diffraction signal if reflection mode is used instead [58] , [59] , [60] , [61] , [62] , [63] , [64] , [65] . The schematic layout of our compact DC-accelerated electron diffraction setup is shown in Fig. 6 . A part of the fundamental (800 nm, 50 fs) output beam from a commercial Ti:sapphire laser system (Coherent) was split into two arms by a beam splitter. Infrared optical pulses were converted to 400 nm pump and 266 nm probe radiation through the second and third harmonic generation nonlinear processes, respectively. The pump light was focused down to a 450-μm spot size at the KI sample, while the 266 nm probe was directed onto a gold photocathode generating ultrashort electron bunches. Photoelectrons were finally accelerated to 90 keV by a DC electric field between the photocathode and anode plates. Photoinduced structural changes inside the material were followed with ~1 ps pulses containing ~10 5 electrons confined to a 120-μm spot in diameter at the ultrathin KI film ( vide infra Sample preparation section below). Diffracted and directly transmitted electrons were focused with the magnetic lens onto a 1:1 fibre-coupled CCD camera (Quad-RO 4320, Princeton Instruments) coated with a P20 phosphor scintillator. The time delay between the photoexcitation and electron pulses was adjusted by changing the optical pump-probe path difference using a motorized translational stage. For single-shot measurements, samples were moved between excitation pulses so that each pump pulse would hit a fresh spot. In contrast to previous studies [66] , [67] on alkali halide materials using high energy (500–600 keV) and high fluence electrons, no structural changes in KI samples were observed during electron beam irradiation with more than 200 consecutive 90 keV electron pulses. 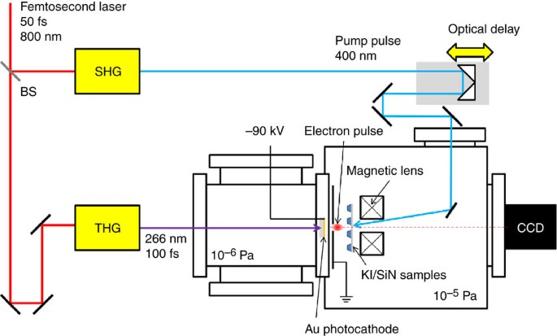Figure 6: Schematic diagram of the FED setup. BS, beam splitter; CCD, charge-coupled device camera; SHG, second harmonic generation; THG, third harmonic generation. Figure 6: Schematic diagram of the FED setup. BS, beam splitter; CCD, charge-coupled device camera; SHG, second harmonic generation; THG, third harmonic generation. Full size image Single-shot fs optical reflectivity measurements Single-shot optical pump-probe experiments were performed in reflection mode on single-crystalline Si, NaCl, CsI and polycrystalline KI films. All samples were photoexcited with 400 nm (3.1 eV) and 70 fs optical pump pulses focused on the target at an incident angle of 30° from the surface normal. Different degrees of photoexcitation conditions were achieved by varying the incident pump laser fluence in the 35–1,100 mJ cm −2 range. The probe infrared (800 nm, 50 fs) or white-light pulses (see Supplementary Fig. 5 ) were focused within the photoexcited area of the sample at a near-Brewster’s incident angle of 60°. In the course of this experiment, pump and probe laser beams were s - and p -polarized, respectively. The reflected signal intensities were registered with a slow photodiode (~100 μs response time) for the infrared probe or using an optical spectrometer (Avantes) when the dynamics were studied with the white-light probe. Single-shot ion detection measurements A simple ion detection system was built to determine the relative ion yield as a function of the incident laser fluence. The system is composed of an extraction electrode aperture with either negative or positive polarity at 2.5 kV with respect to ground potential, a drift tube of 200 mm and a Faraday cup, inside a vacuum chamber. The ions are generated by incident s -polarized 400-nm optical pulses, extracted by the electrode and detected by the Faraday cup. The reflection of the incident 400-nm pulses from the samples is used as a trigger for the ion measurements. An I – V converter is used to record the time-of-flight ion signal in an oscilloscope. The sample is translated between laser shots to make sure that a fresh sample area is exposed to each laser excitation pulse; that is, single-shot photoexcitation conditions were used. Sample preparation Polycrystalline 50-nm- and 100-nm-thick KI films were prepared by thermal deposition on freestanding silicon nitride windows (30 nm thick), and coated with a very thin (<5 nm) carbon layer to protect the KI films from moisture. Thicker and uncoated, 2.5-μm-thick KI films were also prepared and used for time-resolved optical reflectivity and crater depth measurements. The deposition rate and film thickness were monitored in situ with a quartz oscillator. Freestanding silicon nitride windows were produced using conventional anisotropic chemical etching methods. The sample crystallinity of KI films was characterized with static X-ray diffraction and electron diffraction. 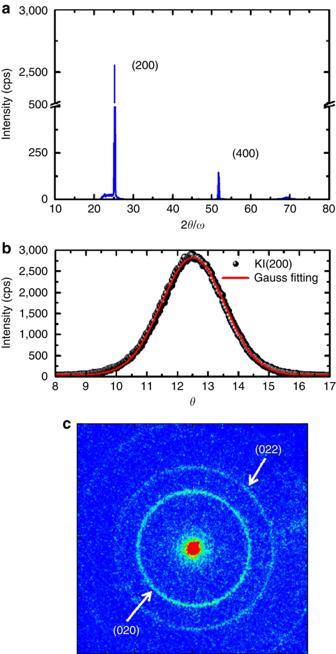Figure 7: Characterization of KI thin film crystallinity. (a) X-ray diffraction spectrum from KI samples. (b) X-ray rocking curve for the reflection from KI (200) plane. (c) Electron diffraction pattern from a 50-nm-thick KI film. Figure 7a shows the X-ray diffraction spectrum from the KI sample. The diffraction lines from KI (200) and (400) lattice planes are observed, suggesting that crystallites are longitudinally oriented in the ‹100› direction. This conclusion is also supported by the rocking curve measurement shown in Fig. 7b . The single-crystalline Si, NaCl and CsI samples were used for the experiments as purchased. Out of numerous attempts to prepare thin crystalline samples from different alkali halides under various deposition conditions, films from KI were the only ones with good crystallinity for single-shot FED experiments. To the best of our knowledge, there are also no commercial suppliers providing single-crystalline KI samples. Figure 7: Characterization of KI thin film crystallinity. ( a ) X-ray diffraction spectrum from KI samples. ( b ) X-ray rocking curve for the reflection from KI (200) plane. ( c ) Electron diffraction pattern from a 50-nm-thick KI film. Full size image Computational method The potential energy curves of the lowest two 1Σ + states of the NaCl molecules were calculated using the multi-state, multi-reference CASPT2 (MS-MR-CASPT2) method as implemented in the MOLPRO 2012.1 computational chemistry software package. The cc-pCVDZ and aug-cc-pCVDZ basis sets were used for the metal atoms and the halogen atoms, respectively. For the NaCl molecule, the active orbitals were: 7σ, 8σ, 9σ, 10σ, 3π x , 4π x , 3π y and 4π y , that is, an active space of eight electrons in eight orbitals. All orbitals were included in the perturbation calculation. The potential energy curves are presented in Supplementary Fig. 6 . The equilibrium metal–halogen distance on the 1 1 Σ + curve is 2.421 Å. The avoided crossing between the 1 1 Σ + and 2 1 Σ + states is found at a distance of 7.8 Å. How to cite this article: Hada, M. et al. Cold ablation driven by localized forces in alkali halides. Nat. Commun. 5:3863 doi: 10.1038/ncomms4863 (2014).